Moderate doping leads to high performance of semiconductor/insulator polymer blend transistors Polymer transistors are being intensively developed for next-generation flexible electronics. Blends comprising a small amount of semiconducting polymer mixed into an insulating polymer matrix have simultaneously shown superior performance and environmental stability in organic field-effect transistors compared with the neat semiconductor. Here we show that such blends actually perform very poorly in the undoped state, and that mobility and on/off ratio are improved dramatically upon moderate doping. Structural investigations show that these blend layers feature nanometre-scale semiconductor domains and a vertical composition gradient. This particular morphology enables a quasi three-dimensional spatial distribution of semiconductor pathways within the insulating matrix, in which charge accumulation and depletion via a gate bias is substantially different from neat semiconductor, and where high on-current and low off-current are simultaneously realized in the stable doped state. Adding only 5 wt% of a semiconducting polymer to a polystyrene matrix, we realized an environmentally stable inverter with gain up to 60. Conjugated polymers are the subject of intensive research and development, as they promise large area fabrication of semiconductor devices via low-temperature solution processing. With regard to organic field-effect transistors (OFETs), tailoring the conjugated backbone [1] , [2] , [3] , [4] , [5] , [6] , [7] , [8] , [9] , [10] and the side-chain architecture [11] , [12] , [13] , and optimizing the layer morphology [14] , [15] , [16] , [17] , [18] , [19] , [20] raised the performance of these materials to values comparable to that of amorphous silicon, with mobilities in excess of 0.1 cm 2 V −1 s −1 . However, for a widespread application of these devices, air stability and material costs are important features that need to be improved. Blends of semiconducting and insulating polymers have recently been shown to exhibit reasonably high mobilities and on/off ratios [21] , [22] , [23] , [24] , [25] , [26] , [27] , [28] , often exceeding the corresponding values measured for pure layers of the semiconducting polymers. As high performance could be realized even for a low concentration of the active semiconductor component mixed into an inert polymer matrix, these blends allow a fine tuning of the active layer’s rheological and optical properties without compromising charge transport. This property triggered intense research on the structural and electrical properties of the active blend layer. Improved performance of the blends with mobility up to 0.1 cm 2 V −1 s −1 has been attributed to an enhanced crystallinity of the conjugated polymer in the blend [24] and/or enrichment of the conjugated polymer at the polymer film/dielectric interface [24] , [25] or the film/vacuum surface [26] . In addition, some of these blend OFETs exhibit superior stability in air, and this stability was mainly ascribed to the encapsulation of the active component [25] . However, a consistent picture explaining the superior performance and stability of these blends is still missing. Here, via doping, we show a drastic improvement in transistor performance of composites comprising a low concentration of benchmark semiconductor polymers incorporated in an insulating polymer matrix. Our work not only illuminates the general mechanism leading to stable device performance of semiconductor/insulator polymer composites, but also proposes doping of conjugated polymers within an insulating matrix as a new approach to substantially promote its OFET performance. Doping in diluted air We found that blends of poly(3-hexylthiophene) (P3HT) [14] , [29] , [30] with polystyrene (PS; blended in a 0.05/0.95 ratio) measured immediately after preparation had a surprisingly poor performance. Spincoating of these blends was performed in glovebox atmosphere (N 2 , ~1 p.p.m. oxygen and water), followed by annealing in vacuum (to remove residual volatile solvent, impurities or dopant molecules) and evaporation of gold source/drain contacts in high vacuum (see Methods). We assume that this procedure results in intrinsic (non-doped) materials. The performance of these blends improved rapidly when kept in a nitrogen glovebox atmosphere with low concentrations of oxygen and water (both ca. 1 p.p.m. ), saturating after 1 day at a mobility of 0.1–0.2 cm 2 V −1 s −1 and on/off ratios as high as 10 6 . The in-situ ecvolution of the transfer characteristics of such a P3HT/PS blend in a bottom-gate top-electrode transistor configuration ( Fig. 1a ) shows that the on-current increased drastically with time, whereas the off-current barely changed (evolution of output characteristic in ‘diluted air’, see Supplementary Fig. S1 ). The final mobility is about one to two orders of magnitude higher than in neat P3HT, either on non-treated SiO 2 or on SiO 2 treated with hexamethyldisilazane (HMDS; Fig. 1b and c ). Exposure of a P3HT/PS (5% P3HT) blend directly to air (humidity 33%) for 1 h had the same effect as storage in N 2 glovebox atmosphere for 1 day. 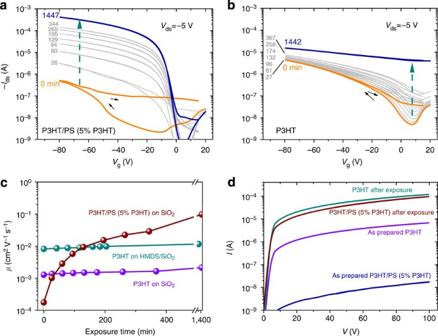Figure 1: The effect of doping on the transistor performance of P3HT/PS blends and neat P3HT. (a,b)In-situevolution of the transfer characteristics (Vds=−5 V, linear regime) on exposure time in ‘dilute air’ (N2atmosphere with O2concentration ~1 p.p.m. and H2O ~1 p.p.m.). P3HT/PS (5% P3HT) (a) (on bare SiO2); neat P3HT (b) (on bare SiO2). The exposure time for each transfer curve was shown. (c) Dependence of the hole mobility (μlin) on exposure time for P3HT/PS (5% P3HT) (on bare SiO2) and neat P3HT (on bare SiO2and HMDS-coated SiO2, respectively).μlinwas extracted from the transfer characteristics atVds=−5 V. (d)In-situ I–Vcurve evolution of films on glass substrates (electrode distance 100 μm, electrode length 14.85 cm) in N2atmosphere with O2~5 p.p.m. and H2O ~1 p.p.m.), which shows more drastic increase of conductance of P3HT/PS (5% P3HT) film as compared with neat P3HT. The exposure times for P3HT/PS (5% P3HT) and P3HT film are 151 and 149 min, respectively, ind, and the conductance does not increase any more with longer exposure time under this condition. Figure 1: The effect of doping on the transistor performance of P3HT/PS blends and neat P3HT. ( a , b ) In-situ evolution of the transfer characteristics ( V ds =−5 V, linear regime) on exposure time in ‘dilute air’ (N 2 atmosphere with O 2 concentration ~1 p.p.m. and H 2 O ~1 p.p.m.). P3HT/PS (5% P3HT) ( a ) (on bare SiO 2 ); neat P3HT ( b ) (on bare SiO 2 ). The exposure time for each transfer curve was shown. ( c ) Dependence of the hole mobility ( μ lin ) on exposure time for P3HT/PS (5% P3HT) (on bare SiO 2 ) and neat P3HT (on bare SiO 2 and HMDS-coated SiO 2 , respectively). μ lin was extracted from the transfer characteristics at V ds =−5 V. ( d ) In-situ I – V curve evolution of films on glass substrates (electrode distance 100 μm, electrode length 14.85 cm) in N 2 atmosphere with O 2 ~5 p.p.m. and H 2 O ~1 p.p.m. ), which shows more drastic increase of conductance of P3HT/PS (5% P3HT) film as compared with neat P3HT. The exposure times for P3HT/PS (5% P3HT) and P3HT film are 151 and 149 min, respectively, in d , and the conductance does not increase any more with longer exposure time under this condition. Full size image For the neat P3HT devices, exposure to glovebox atmosphere has a dramatically different impact ( Fig. 1b ), causing a minor increase in mobility ( Fig. 1c ) but mainly increasing the off-current and shifting the threshold voltage to positive values, which is indicative of unintentional p-type doping at low-to-moderate doping ratios [31] , [32] , [33] , [34] . From conductivity measurements on neat films and blend films with a two-terminal device on a glass substrate, we observe a progressive increase in current, with both layers reaching similar conductivities after prolonged exposure ( Fig. 1d ). Comparing the conductivity of the neat P3HT (ca. 10 −4 S cm −1 ) with that of electrochemically or molecularly doped P3HT [33] , [34] , we estimate a doping concentration of ca. 0.1% of total P3HT monomers, which we denote ‘moderate doping’ in the following. We can therefore conclude that in our case the increase in performance of the blend OFET is determined by the unintentional doping of the P3HT in the blend, following a different mechanism from the one reported recently for the rather high stability of some conjugated materials/polymer systems [25] , where the improved stability was interpreted in terms of ‘encapsulation’ of the semiconducting polymer by the insulating component, preventing oxygen from penetrating deeply into the layer [25] . The high conductance of P3HT/PS (5% P3HT), and the low off-current as well as its stable threshold voltage as shown in Fig. 1 , implies that the transistor switching mechanism of the blend is different from that of neat P3HT. Molecular dopants and different semiconducting polymers To check the role of doping and the universality of the mechanism, we performed extensive studies on transistors with molecular doping and on blends containing other high-performance active polymers. 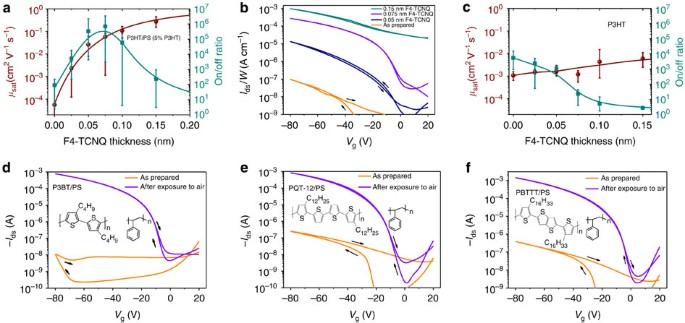Figure 2: Blend transistors with intentional doping or air-exposed transistors comprising different high-performance conjugated polymers. (a) Dependence of mobility and on/off ratio of a P3HT/PS (5% P3HT) blend transistor on the nominal thickness of F4-TCNQ deposited on top of the blend. (b) Transfer characteristics of blend transistors for selected F4-TCNQ layer thicknesses. (c) Dependence of mobility and on/off ratio of a neat P3HT transistor on the thickness of F4-TCNQ deposited on top of the semiconductor. (d–f) Transfer characteristics of as-prepared and air-exposed blend FETs using three different high-performance semiconducting polymers (5% semiconductor polymer in PS; spincoating at 80 °C). Froma–f,Vds=−100 V. (a,c) Error bars are derived from measurements on at least three devices for each case. Figure 2a summarizes performance data of P3HT/PS (5% P3HT) transistors, where the active channel was covered with an ultra-thin layer of tetrafluoro-tetracyanoquinodimethane (F4-TCNQ), which has been shown to be an efficient molecular p-dopant for P3HT [34] , [35] . A P3HT concentration of 5% has been chosen as the composition has the highest mobility upon doping in air ( Supplementary Fig. S2 ). We found that both the mobility and the on/off ratio of the blend transistors improve rapidly when increasing the F4-TCNQ layer nominal thickness to ca. 0.1 nm, because the on-current increases faster than the off-current. Further addition of the p-dopant leads to a decrease of the on/off ratio, probably as a result of over-doping, whereas the mobility still increases slowly. In contrast, neat P3HT covered with F4-TCNQ undergoes a continuous decrease of the on/off ratio with increasing F4-TCNQ nominal layer thickness ( Fig. 2c ), a situation that is similarly encountered in air-exposed neat P3HT and attributed to the expected doping-induced increase of bulk conductivity combined with a positive shift of threshold voltage. Figure 2: Blend transistors with intentional doping or air-exposed transistors comprising different high-performance conjugated polymers. ( a ) Dependence of mobility and on/off ratio of a P3HT/PS (5% P3HT) blend transistor on the nominal thickness of F4-TCNQ deposited on top of the blend. ( b ) Transfer characteristics of blend transistors for selected F4-TCNQ layer thicknesses. ( c ) Dependence of mobility and on/off ratio of a neat P3HT transistor on the thickness of F4-TCNQ deposited on top of the semiconductor. ( d – f ) Transfer characteristics of as-prepared and air-exposed blend FETs using three different high-performance semiconducting polymers (5% semiconductor polymer in PS; spincoating at 80 °C). From a – f , V ds =−100 V. ( a , c ) Error bars are derived from measurements on at least three devices for each case. Full size image We also found that similar phenomena occur in blends of other conjugated polymers ( Table 1 and Fig. 2d–f ), such as poly(3-butylthiophene) (P3BT) [29] , [36] , [37] , poly(3,3′′′-didodecylquaterthiophene) (PQT-12) [2] , [38] and poly(2,5-bis(3-hexadecylthiophen-2-yl)thieno[3,2-b]thiophenes) (PBTTT) [3] , blended with PS or poly(methylmethacrylate) (PMMA). This demonstrates that the observed effect is rather general to thiophene-based high-performance semiconducting polymers blended at low concentration with an insulator. Remarkably, the air-exposed PQT-12/PS or PBTTT/PS blends have lower mobilities than P3HT/PS, probably because the degree of doping via exposure to air is smaller for PQT-12 or PBTTT; this is consistent with reports that neat PQT-12 and PBTTT are more stable to air exposure than neat P3HT [2] , [3] . However, F4-TCNQ is able to dope PQT-12 and PBTTT efficiently. Blends of both polymers with PS, covered by less than 5 Å F4-TCNQ, gave mobilities higher than 0.1 cm 2 V −1 s −1 combined with reasonable on/off ratios. We further noted that transistors of these blends with a F4-TCNQ thickness above 5 Å missed a distinct saturation plateau in the output characteristics and suffered from low on/off ratio, but their normalized transconductance g m / W ( g m =d I ds /d V g , where W is the channel width) was very high, up to 40–60 μS cm −1 ( Table 1 and Supplementary Fig. S3 ). Table 1 Doping induced improvement of OFET performance using different semiconductor/insulator polymer blends and doping methods. Full size table Morphology requirement for low off-current While the performance of the undoped layer in the blend semiconductor is very poor, and doping mainly increases the mobility in the on-state without a noticeable increase of the off-current, doping the neat layers has an only weak effect on the on-current but increases substantially its off-current. This behaviour must then be related to the particular morphology of our blends. To this end, we used incremental O 2 plasma etching in combination with ultraviolet–visible absorption spectroscopy to obtain information on the vertical composition profile. The spectra in Fig. 3a show that for the P3HT/PS (5% P3HT) blend spincoated on SiO 2 , most of the P3HT is enriched at the top part of the film. This is in agreement with our grazing incidence X-ray diffraction measurements in which incidence angles were chosen to probe just the surface region and the entire film, respectively ( Supplementary Fig. S4 ). The surface-sensitive scan shows a clear enhancement in intensity for diffraction peaks, which can be attributed to P3HT. However, a small amount of crystalline P3HT (as characterized by a broad absorption with peaks at ca. 560 and 610 nm) is embedded in the PS matrix, even 10 nm below the surface ( Fig. 3a ). X-ray photoemission spectroscopy (XPS) on P3HT/PS (5% P3HT) revealed a vertical composition gradient with a P3HT content of ca. 30% at the top surface and no P3HT at the interface to the SiO 2 dielectric ( Supplementary Fig. S5 ). Our ultraviolet–visible spectroscopy and XPS data suggest a morphology where the topmost layer does not consist exclusively of conjugated polymer chains and where semiconducting material also penetrates the bulk of the blend. Transmission electron microscopy (TEM) images ( Fig. 3b and Supplementary Fig. S6 ) imply the typical characteristic size of P3HT crystallites in the blend to be less than 100 nm. Atomic force microscopy (AFM) measurements confirmed that spincoated P3HT/PS films with only 5% P3HT display a rather homogenous lateral morphology at the micrometre scale ( Supplementary Fig. S7 ). These findings suggest that the film consists of a connected network of nanometre-scale crystallites. This morphology for P3HT/PS (5% P3HT) is schematically shown together with a top-contact transistor configuration as an inset in Fig. 3c . 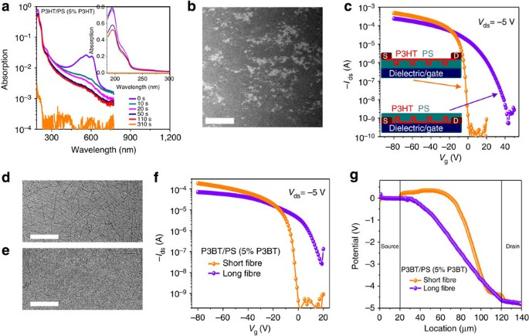Figure 3: The relationship between performance of air-exposed transistor and film morphology. (a) Ultraviolet–visible absorption spectroscopy of P3HT/PS (5% P3HT) film after different times of etching by oxygen plasma. Inset is a linear plot of the main graph. (b) Dark-field TEM of P3HT/PS (5% P3HT) film showing P3HT forms nanometre-scale crystallites. (c) Transfer curves of air-doped P3HT/PS (5% P3HT) film with as-spincoated and inverted morphology. The schemes in the insets were confirmed by O2plasma etching in combination with ultraviolet–visible absorption spectroscopy (a) and TEM (b). (d,e) Bright-field TEM of P3BT/PS (5% P3BT) film spincoated at 22 and 80 °C, which yield different lengths of P3BT fibres. (f) Transfer curves of air-doped P3BT/PS (5% P3BT) film with different fibre lengths. (g) Surface potential profile (Vg=0 V andVds=−5 V) across the transistor channel of air-doped P3BT/PS (5% P3BT) film with different fibre lengths. The scale bars inb,dandeare 1 μm. Figure 3: The relationship between performance of air-exposed transistor and film morphology. ( a ) Ultraviolet–visible absorption spectroscopy of P3HT/PS (5% P3HT) film after different times of etching by oxygen plasma. Inset is a linear plot of the main graph. ( b ) Dark-field TEM of P3HT/PS (5% P3HT) film showing P3HT forms nanometre-scale crystallites. ( c ) Transfer curves of air-doped P3HT/PS (5% P3HT) film with as-spincoated and inverted morphology. The schemes in the insets were confirmed by O 2 plasma etching in combination with ultraviolet–visible absorption spectroscopy ( a ) and TEM ( b ). ( d , e ) Bright-field TEM of P3BT/PS (5% P3BT) film spincoated at 22 and 80 °C, which yield different lengths of P3BT fibres. ( f ) Transfer curves of air-doped P3BT/PS (5% P3BT) film with different fibre lengths. ( g ) Surface potential profile ( V g =0 V and V ds =−5 V) across the transistor channel of air-doped P3BT/PS (5% P3BT) film with different fibre lengths. The scale bars in b , d and e are 1 μm. Full size image To realize an inverted morphology (with most P3HT at the interface to the gate insulator and some P3HT extending upwards), we spincoated P3HT/PS (5% P3HT) on a glass substrate, and then the film was floated onto deionized water. This layer was picked up from the top with a bottom-gate/bottom-contact transistor configuration (with 300 nm SiO 2 passivated with HMDS). This device architecture and the inverted layer morphology are also shown as an inset in Fig. 3c . Interestingly, such a device showed a large positive shift of the threshold voltage upon doping ( Supplementary Fig. S8 ). As a consequence, the device with a doped inverted layer exhibited a large off-current, indicating insufficient depletion of the conductive pathways at zero bias ( Fig. 3c ). In addition, the rather poor solubility of P3BT [39] , [40] allowed us to control the morphology of the P3BT/PS (5% P3BT) blend by changing the spincoating temperature. As shown in bright-field TEM ( Fig. 3d and e ), the sample prepared at 22 °C from o -dichlorobenzene (a poor solvent for P3BT, which, therefore, crystallizes in solution at 22 °C) consists of a network of interconnected P3BT fibres longer than 1 μm. In contrast, samples spincoated at 80 °C yield smaller P3BT crystals with length typically below 100 nm on average. The two films were denoted by ‘long fibre’ and ‘short fibre’ for clarity in this work. We find that similar to what is reported above for P3HT/PS blends, the performance of undoped P3BT/PS with short fibres is very poor but increases drastically upon exposure to air ( Fig. 2d ). In contrast to this, the mobility of undoped P3BT/PS (5% P3BT) films with long fibres is already on the order of 10 −2 cm 2 V −1 s −1 , and exposure to air does not increase its mobility but reduces the on/off ratio by shifting the threshold voltage towards positive values ( Fig. 3f and Supplementary Fig. S9 ). Surface potential profiles [41] (obtained by scanning Kelvin probe) across the transistor channel of P3BT/PS (5% P3BT) films with different fibre lengths are shown in Fig. 3g . The profile of the short-fibre transistor channel reveals a typical ‘pinch-off’ region near the drain contact at V g =0 V and V ds =−5 V. For the film with long fibres, a resistor-like potential profile is observed, characteristic for a layer with homogeneous ohmic conduction along the entire channel, which is consistent with the observation of a high off-current and poor on/off ratio. Our electrical and structural characterization shows that good and stable performance of blends containing a low concentration of a semiconducting polymer in an insulating polymer matrix requires a specific morphology, with most of the semiconductor forming a poorly interconnected network of crystallites on the top surface (well separated from the dielectric). The fact that doping of these layers causes high currents in the two-terminal device means that the crystallites are connected via long tie chains or amorphous domains. In addititon, some of the semiconducting network penetrates the inert matrix, forming a bulk-distributed semiconductor–insulator interface. This morphology is schematically depicted in Fig. 4a . We propose that applying a positive gate bias will first deplete some of the conjugated domains closest to gate electrode, interrupting the conductive pathways and leading to low off-currents even at moderate doping levels. Alternatively, in the undoped device gate-induced charge accumulation will take place first on conjugated domains that are closest to gate electrode, but this process might screen the formation of space charge in crystallites further away from the gate, thus preventing the formation of a fully conductive network. Owing to the lack of accumulated charge, carrier motion along these upper-lying crystallites will be dominated by trap states [42] . Oxygen-induced doping will increase the charge concentration, creating a continuous conductive network between source and drain. 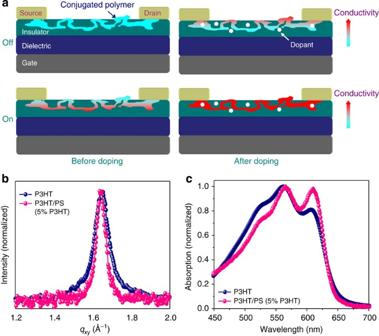Figure 4: Relationship between crystalline ordering and field-effect mobility. (a) Scheme of gate-induced charge accumulation and depletion in the undoped or moderately doped semiconductor/insulator polymer blend in the on and off state. Nanometre-scale crystallites are interconnected at the top part of the film. (b) In-plane (qxyplane) profile of grazing incidence angle x-ray diffraction. The (020) diffraction peaks (after subtracting background), which corresponds to π–π stacking distance, imply better crystalline order of P3HT in PS than in neat P3HT. (c) Light absorption spectra of P3HT and P3HT/PS (5% P3HT) blend film (normalized after subtracting background). Figure 4: Relationship between crystalline ordering and field-effect mobility. ( a ) Scheme of gate-induced charge accumulation and depletion in the undoped or moderately doped semiconductor/insulator polymer blend in the on and off state. Nanometre-scale crystallites are interconnected at the top part of the film. ( b ) In-plane ( q xy plane) profile of grazing incidence angle x-ray diffraction. The (020) diffraction peaks (after subtracting background), which corresponds to π–π stacking distance, imply better crystalline order of P3HT in PS than in neat P3HT. ( c ) Light absorption spectra of P3HT and P3HT/PS (5% P3HT) blend film (normalized after subtracting background). Full size image Origin of the high mobility in the blends Finally, we would like to address the high mobilities of our blends at moderate doping levels, which are well above the values found for the neat semiconducting material. Remarkably, x-ray diffraction ( Fig. 4b ) reveals that the width of the (020) diffraction peak related to the π–π stacking direction of P3HT chains is much narrower [43] in the P3HT/PS (5% P3HT) blend than in neat P3HT, implying a better order of P3HT chain in the PS matrix. Here the coherence length is ~12 nm, as compared with ~7 nm of neat P3HT. We propose that during film drying, the PS matrix is still plasticized by solvent molecules, and that this mobile environment enables the formation of P3HT crystallites with better interchain order [44] , [45] . We also found the 0–0 transition of the P3HT absorption to increase with decreasing P3HT concentration ( Fig. 4c and Supplementary Fig. S10 ). According to the recently published model by Spano and colleagues [46] , [47] , the relative strength of the 0–0 vibronic transition is a direct measure of the intermolecular coupling strength, which is further related to the conjugation length and intrachain order of the interacting chains in the P3HT aggregates. In accordance to this finding, the activation energy describing the temperature dependence of the drain current at accumulation was smaller for the blend ( Supplementary Fig. S11 ), suggesting a better order of P3HT chains within the nanocrystallites in the blend. This is also consistent with larger coherence length as estimated from X-ray scattering. It is noted that a narrower diffraction peak also implies shallower traps [48] , which leads to lower activation energy as well. With a thickness of ~20 nm and a conjugated polymer content of only 5%, these films are virtually transparent and almost colourless ( Supplementary Fig. S10 ), whereas the devices work well under moderate light illumination ( Fig. 5a ). All of these merits open up new opportunities in display applications. We, finally, would like to point out that doping of our semiconductor/insulator polymer blends via exposure to air saturated rapidly, and exposure longer than 1 h did not substantially change the OFET characteristics, implying a good long-term environmental stability of the transistor when stored in air ( Fig. 5b ). This merit is highly desirable for reliable circuits [49] . As an example of successful application of such semiconductor/insulator polymer blends, a digital converter consisting two environmental stable P3HT/PS OFETs showed reliable switching capability with a gain as high as 60 ( Fig. 5c ). 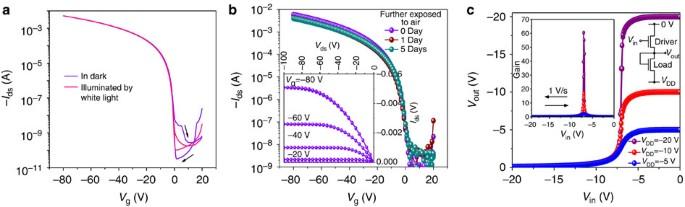Figure 5: Stability of doped semiconductor/insulator polymer blends and its application in circuit prototype. (a) Transfer characteristics (Vds=−100 V) of air-exposed P3HT/PS (5% P3HT) OFET in dark and under moderate illumination (white light, ~5 mW cm−2). (b) Transfer characteristics (Vds=−100 V) of a P3HT/PS (5% P3HT) blend immediately after 1 h exposure to air (0 day, with output characteristics as inset) and after further storage in air for 1 and 5 days (temperature ~22 °C; humidity ~60%). (c) Transfer characteristics of an air-exposed P3HT/PS digital inverter with the gain curve shown in the inset. Figure 5: Stability of doped semiconductor/insulator polymer blends and its application in circuit prototype. ( a ) Transfer characteristics ( V ds =−100 V) of air-exposed P3HT/PS (5% P3HT) OFET in dark and under moderate illumination (white light, ~5 mW cm −2 ). ( b ) Transfer characteristics ( V ds =−100 V) of a P3HT/PS (5% P3HT) blend immediately after 1 h exposure to air (0 day, with output characteristics as inset) and after further storage in air for 1 and 5 days (temperature ~22 °C; humidity ~60%). ( c ) Transfer characteristics of an air-exposed P3HT/PS digital inverter with the gain curve shown in the inset. Full size image Here, for a class of blends comprising a low concentration of benchmark semiconductor polymers incorporated in insulator polymer matrices, we show that doping is necessary to achieve high on-currents, and that in contrast to transistors with doped layers of the neat semiconducting polymers, such doped blend transistors exhibit very high on/off ratios. We identified a morphology feature enabling this behaviour, namely nanometre-scale semiconductor domains and a vertical composition gradient as a result of incomplete phase segregation. A semiconductor-enriched top layer together with a lower concentration of semiconductor in the bulk insulating matrix enables a quasi three-dimensional spatial distribution of semiconductor pathways within the insulating matrix. The minority semiconductor domains closer to the gate have a crucial role in the performance of the doped device. Therefore, in such a morphology, charge accumulation and depletion via a gate bias is substantially different from the neat semiconductor, leading to high on-current and low off-current in the (moderately) doped state. With such transistors, we achieved an environmentally stable digital inverter with gain up to 60. Our work not only demonstrates a general mechanism leading to good and stable device performance of polymer blends with a very low concentration of the semiconducting component, but also proposes guidelines for the development of high-performance transistors using doped semiconducting polymers embedded within an insulating matrix. This new approach promotes the OFET performance while providing a simple fabrication process. With this guidance, highly transparent transistors with field-effect mobilities comparable to that of amorphous silicon, combined with environmental stability and mechanical robustness, might become feasible. Materials P3HT (98% head-to-tail regioregularity, M w =32 kDa, PDI=2.4, Sepiolid P200, BASF); P3BT (97% head-to-tail regioregularity, M w =39 kDa, PDI=2.3, Rieke Metals, Inc.); PQT-12 ( M w =27 kDa, PDI=1.7, supplied by Professor Ullrich Scherf); PBTTT (PBTTT–C16, M w =48 kDa, PDI=1.9, FN3814, Merck Chemicals Ltd); amorphous PS ( M w =95 kDa, PDI =1.1, Fluka AG); amorphous PMMA ( M w =40 kDa, PDI =1.2, Fluka AG); F4-TCNQ (Tokyo Kasei Kogyo Co., Ltd (TCI)). Sample preparation To get a well-defined pristine state (undoped state), all sample preparation procedures were performed in a nitrogen-filled glovebox if not stated otherwise. All polymers in this work were dissolved in solvent o -dichlorobenzene with a concentration of 8 mg ml −1 individually. For P3BT, PQT-12 and PBTTT, elevated temperature ~100 °C was used for dissolution. Samples were prepared by spincoating either a solution of the pure semiconducting polymer, or the semiconductor polymer solution mixed with a solution of the insulating polymer in the desired ratio. For OFET preparation, the polymer solution was spincoated on n-doped silicon covered with 300 nm thick SiO 2 layer, which had been precleaned using water, acetone and isopropanol in this sequence. The sample was subsequently heated in vacuum at 140 °C for 10 min in a vacuum oven placed in the glovebox, to dissipate residual solvent/impurity and versatile dopants. Top-contact bottom-gate OFET devices were finally completed by evaporating ~100 nm gold source/drain electrodes in vacuum at pressure below 10 −6 mbar after purging for more than 3 h (to further dissipate the residual volatile dopant). After evaporation, the device was kept in vacuum (below 10 −6 mbar) for 0.5 h to cool down the samples that had been inevitably heated during evaporation. Note that the evaporator is directly placed within a nitrogen-filled glovebox (with both O 2 and H 2 O concentration around 1 p.p.m.). For molecular doping, F4-TCNQ was deposited by thermal evaporation in vacuum (base pressure 10 −6 mbar) directly onto the active polymer film. For inverted morphology, with most P3HT at the interface to the gate insulator and some P3HT extending upwards, the P3HT/PS (5% P3HT) film was spincoated on glass substrate and then was floated onto deionized water. This layer was picked up from the top with a bottom-gate bottom-contact transistor configuration (with 300 nm SiO 2 passivated with HMDS). Output and transfer characteristics were recorded in glovebox (includes the air-doped devices) using an Agilent 4155C semiconductor parameter analyser. μ sat from saturation region were calculated according to I ds = (WC i /2 L)μ sat (V g − V 0 ) 2 , where I ds is the source-drain current; C i (11.9 nF cm −2 ) is the capacitance per unit area; L (100 μm) is the channel length; W is the channel width, which is 148.5 mm for pristine/air-exposed devices and varies from 1 to 148.5 mm for F4-TCNQ-doped devices (note that the on-current for different doping level varies drastically, up to >6 orders magnitude, so we use smaller W for doped device and larger W for non-doped devices, to extract reliable device parameters); V g and V 0 are gate voltage and extrapolated threshold voltage, respectively. μ lin from linear region were calculated according to I ds = (WC i /L)μ lin (V g – V 0 – V ds /2 )V ds . On/off ratios were estimated in terms of I ds ( V g =−80 V)/ I ds ( V g = V on , which is the onset voltage) from the transfer characteristics. In the cases where the transistor did not switch off in the considered voltage range, we used I ds ( V g =80 V) as the off-current. Although most transistors were fabricated by spincoating the polymer onto bare SiO 2 , transistors with passivated SiO 2 surfaces were also studied for comparison. After the SiO 2 surface was thoroughly cleaned with solvents and had undergone oxygen plasma treatment (5 min at a power of 200 W), the sample was exposed to HMDS-saturated vapour for 8 h at 80 °C. Afterwards, the active polymer material was spincoated from chloroform (10 mg ml −1 ). Film characterization AFM measurements were performed on a Multimode Atomic Force Microscope (Veeco Metrology) in air. AFM images were collected using tapping mode. Surface potential profile within OFET was performed in air on a commercial Solver SPM (NT-MDT, Russia) equipped with an optical microscope. Kelvin mode was used to simultaneously acquire topography and potential contrast. TEM images were recorded using a TECNAI G2 TEM setup at an acceleration voltage of 200 kV. The films for TEM measurements were peeled up directly from the transistor devices through exposure of the device to hydrofluoric acid vapour for ca. 1 s. Afterwards, the films were floated onto deionized water. The polymer films were then picked up using copper grid without any supporting film. The ultraviolet–visible spectrum was collected on a VARIAN Cary 5000 UV–vis-NIR Spectrophotometer and Lambda 950 Spectrometer (PerkinElmer). The samples were prepared upon spincoating on glass/fused-glass substrate, under the same preparation conditions as device fabrication. To get the vertical composition profile, we used incremental O 2 plasma (power 30 W, O 2 pressure 0.1 mbar) etching in combination with ultraviolet–visible absorption spectroscopy. The films for XPS measurements were peeled up from the transistor devices through exposure of the device to hydrofluoric acid vapour for ca. 1 s. Afterwards, the P3HT/PS film was floated onto deionized water. The polymer films were picked up using induim tin oxide (ITO) substrate, from either above or beneath the floated film. In such a case, the top surface (P3HT/PS-vacuum interface) and bottom surface (P3HT/PS-SiO 2 interface) of the original film can be measured by XPS. Grazing incidence angle X-ray diffraction was conducted at Stanford Synchrotron Radiation Lightsource on beamline 11–3. Films were spincoated on SiO 2 , and the grazing incidence angle was 0.1° for coherence length measurements. Incidence angles of 0.08° and 0.12° were used to measure diffraction arising from approximately the top 10 nm and the entire film thickness, respectively. How to cite this article: Lu, G. et al. Moderate doping leads to high performance of semiconductor/insulator polymer blend transistors. Nat. Commun. 4:1588 doi: 10.1038/ncomms2587 (2013).